The statistical geometry of transcriptome divergence in cell-type evolution and cancer In evolution, body plan complexity increases due to an increase in the number of individualized cell types. Yet, there is very little understanding of the mechanisms that produce this form of organismal complexity. One model for the origin of novel cell types is the sister cell-type model. According to this model, each cell type arises together with a sister cell type through specialization from an ancestral cell type. A key prediction of the sister cell-type model is that gene expression profiles of cell types exhibit tree structure. Here we present a statistical model for detecting tree structure in transcriptomic data and apply it to transcriptomes from ENCODE and FANTOM5. We show that transcriptomes of normal cells harbour substantial amounts of hierarchical structure. In contrast, cancer cell lines have less tree structure, suggesting that the emergence of cancer cells follows different principles from that of evolutionary cell-type origination. The number of recognizable cell types varies between metazoan lineages by at least two orders of magnitude, from five in the primitive metazoan Trichoplax to at least 500 in humans [1] , [2] , [3] . The processes that create this diversity, however, are not well understood. The only published model for cell-type origination we are aware of is the so-called sister cell-type model [4] . The model suggests that novel cell types arise through sub-specialization of an ancestral cell type. As a consequence, new cell types arise in pairs, so-called sister cell types. Sister cell types are expected to have more similar gene expression profiles than each of them compared with other cell types, because they initially share most of the developmental pathway of their ancestral cell type. This model thus predicts that the transcriptomes of cell types in one species has substantial amounts of tree structure. An alternative model is that novel cell types arises through the recruitment of co-regulatory modules, recruited from unrelated cell types. Similarly, a new cell type could arise by ‘fusion’ of gene regulatory networks of two unrelated cell types. In either case, the resulting cell types would not be expected to harbour substantial amounts of tree structure. Here we present a statistical tool that allows us to assess the amount of tree structure in a set of cell-type transcriptomes and apply this tool to two data set of cell-type transcriptomes, ENCODE and FANTOM5. We find that the transcriptomes of normal cell types have substantial amounts of tree structure, consistent with the sister cell-type model. In contrast, cancer cells do not retain strong similarities with their cell types of origin, suggesting a different mode of transcriptome divergence in cancer progression than during evolutionary origin of novel cell types. Approach to data analysis In our analysis, we quantify RNA expression profiles from ENCODE Illumina sequencing [5] in terms of tpm (transcripts per million transcripts) based on the frequency of RNA sequencing (RNA-seq) reads mapped to a genomic feature [6] . The FANTOM5 data [7] is from CAGE (Cap Analysis Gene Expression) sequences and is quantified as tags per million, which is quantitatively equivalent to tpm based on Illumina RNA-seq. Thus, we call all RNA abundance measures tpm . We then discretize the tpm of each gene from ENCODE data using an operational threshold of tpm =3, where genes with tpm >3 are coded as expressed (1) and those with tpm ≤3 coded to be not expressed (0; ref. 8 ). This approach is justified by a statistical model of transcript abundance as well as by correlation with chromatin immunoprecipitation data of active chromatin marks [9] . For the FANTOM5 data, an expression threshold of ≥2 tags per million is used, and the results are robust with respect to different thresholds. The rational to focus on qualitative expression profiles is that the exact expression levels of the genes are not a cell-type-specific property but influenced by many environmental and experimental factors. After discretization, each sample is represented as a 0–1 vector of expressed and non-expressed genes ( Fig. 1a ). The similarity of gene expression profiles can be measured as Hamming distance H xy , that is, the number of genes at which the expression state differs for cells x and y . The Hamming distances for all pairs of cell types determine a distance matrix for those samples ( Fig. 1b ). As mentioned above, the sister cell-type model predicts that gene expression profiles of the samples has substantial tree structure or, mathematically, the distance matrix of gene expression profile satisfies the four-point condition [10] (see below). Here we present a statistical test for endogenous ‘treeness’ for gene expression data. 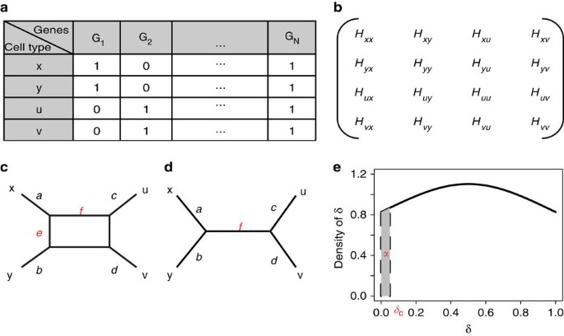Figure 1: The logic of the treeness test. (a) Discretized expression data is represented in a 0–1 matrix where rows represent samples and columns represent genes. The entry is 0 if the gene is not expressed in a particular cell sample and 1 if it is expressed above threshold. (b) The data in the matrix can be represented as a Hamming distance matrix, where each entry is the number of genes where two cell types have different expression values. (c) Any collection of Hamming distances among four samples can be represented in a box graph, which consists of a internal box with dimensionseandf, and terminal branches with lengtha,b,candd. (d) A tree is a special case of a box diagram where one and only one of the inner edges have zero length;e=0 andf>0. (e) Probability density ofδfor random matrices. This distribution is relatively flat with a maximum atδ=0.5. The integral fromδ=0 toδcis the type I error probabilityαfor rejecting the null hypothesis, that is, the probability that aδvalue of ≤δcis due to chance. Figure 1: The logic of the treeness test. ( a ) Discretized expression data is represented in a 0–1 matrix where rows represent samples and columns represent genes. The entry is 0 if the gene is not expressed in a particular cell sample and 1 if it is expressed above threshold. ( b ) The data in the matrix can be represented as a Hamming distance matrix, where each entry is the number of genes where two cell types have different expression values. ( c ) Any collection of Hamming distances among four samples can be represented in a box graph, which consists of a internal box with dimensions e and f , and terminal branches with length a , b , c and d . ( d ) A tree is a special case of a box diagram where one and only one of the inner edges have zero length; e =0 and f >0. ( e ) Probability density of δ for random matrices. This distribution is relatively flat with a maximum at δ =0.5. The integral from δ =0 to δ c is the type I error probability α for rejecting the null hypothesis, that is, the probability that a δ value of ≤ δ c is due to chance. Full size image Tree structure of distance matrices has been investigated extensively in the field of statistical geometry [10] , [11] . If a distance matrix is to be precisely described by a tree, it should satisfy the four-point condition. That is, for any four samples (tetrad) x , y , u , v , with their pairwise distances H ij , the two largest values of H xy + H uv , H xu + H yv and H xv + H yu should be the same ( Fig. 1d ). More generally, distance matrix of any tetrad can be represented in a box graph ( Fig. 1c ). Trees are limiting cases of box graphs, that is, a tree is a box graph in which one and only one of the inner edges is of zero length. Let the inner edges of the box graph be e and f , then the measure of treeness is the so-called delta statistic, δ = e / f , e ≤ f , which can be calculated directly from the distances [11] . For example, the tetrad in fig. 1c , we have H xy + H uv ≤ H xu + H yv ≤ H xv + H yu , so δ is defined as δ -Values close to zero indicate that the distance data conforms to the constraints of a tree. In contrast, δ -values close to 1 are indicative of complete lack of tree structure. Below we will present a statistical model that predicts the probability that a δ -value of less than a certain value δ c is caused by chance. Hence we will calculate the probability that a tetrad from a random 0–1 matrix has a δ -value smaller than a given value, δ≤δ c . This probability can be interpreted as type-I error probability, α , for the null hypothesis that the distance matrix is random. Note that this approach specifically tests only one class of deviations from randomness, namely non-random with respect to ‘treeness’. Significant tree structure requires very low δ -values Preliminary analysis of transcriptomic data suggests that ~40% of mapped genes fulfill the operational criterion of being expressed in any one cell type. Hence, there is a high chance of random similarities among gene expression profiles. We calculated the probability density of the δ -statistic, assuming that the expected proportion of expressed genes in each cell type is r , where r is neither close to 0 nor to 1 (with N being the total number of genes considered). We further assume that the expression indicator of each gene in each cell type is distributed as identical, independent Bernoulli variables with ‘success’ probability r . For a genome with large-enough N and moderate expression rate r , we arrived at an asymptotic null hypothesis distribution independent of N and r , as shown in Fig. 1e and below. The distribution for the δ statistic is quite close to uniform on the unit interval with a maximum at δ =0.5. We then calculated, by direct integration of equation (2), the probability for δ to be smaller than a given threshold δ c . This probability can be interpreted as the type-I error probability for rejecting the null-hypothesis of random structure. This probability is , with the asymptotic solution For a significance level of α =0.05, δ has to be smaller than 0.0587. Transcriptomes of normal cells have extensive tree structure We applied our statistical test to all normal human cell types from the ENCODE RNA-seq data. We obtained read files from 24 samples representing 12 non-cancerous cell types, including fibroblasts, embryonic stem cells, immune cells and others ( Supplementary Table 1 ). We mapped the data and quantified gene expression levels, and converted the data into operationally defined gene expression indicators as expressed and non-expressed. A Hamming distance matrix was calculated and the 24 samples were arranged into 7,740 tetrads, with replicates from the same cell type deliberately avoided. Based on the null distribution (equation (3)) each of the tetrads was assigned an α -value for the treeness test. The distribution of all 7,740 α -values was analysed according to the methods of Benjamini and Hochberg ( Fig. 2a ) [12] , [13] . With this method, it is possible to estimate the number of tetrads that are truly conforming to the null hypothesis, even though one cannot identify them individually. From this α -value distribution, we calculated the fraction of true null hypotheses π 0 =0.33. The value π 0 =0.33 implies that 1− π 0 =0.67 is the fraction of tetrads that actually have tree structure. To estimate the confidence interval for this estimate, we performed a jack-knife procedure yielding a 95% confidence interval of (0.57, 0.77). In other words, 67±10% of the tetrads reflect non-random tree structure, suggesting strong evidence for tree structure among the majority of cell types. 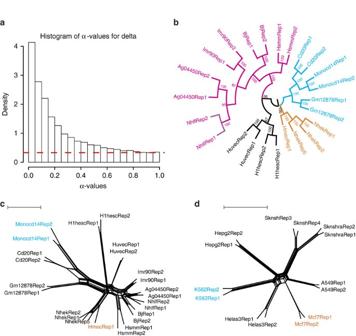Figure 2: Treeness tests on ENCODE data. (a) Distribution ofα-values (significance values) of the treeness test for all tetrads from the 12 normal cell types in the ENCODE data. The high mode nearα=0 indicates that there is a large number of tetrads where the null hypothesis is false, that is, where the tetrad has true tree structure. From this distribution, one can calculate that 100*(1−π0)=67% of the tetrads have true tree structure. (b) Tree relationship among normal cell types based on discretized transcriptomic data using maximum parsimony method21. Colours indicate different groups of cells. Magenta: fibroblast and myoblast cells; cyan: immune cells; orange: epithelial cells; black: others. (c) Neighbour net22,23for the distance matrix for normal cells. Scale bar, 1,000. (d) Neighbour net of the distance matrix for neoplastic cells. Scale bar, 1,000. Note that the cancer cells have a greatly less resolved tree than normal cells, which is also reflected in the treeness statistic. Colour-marked samples are used for treeness test among cancer origin pairs. Figure 2: Treeness tests on ENCODE data. ( a ) Distribution of α -values (significance values) of the treeness test for all tetrads from the 12 normal cell types in the ENCODE data. The high mode near α =0 indicates that there is a large number of tetrads where the null hypothesis is false, that is, where the tetrad has true tree structure. From this distribution, one can calculate that 100*(1− π 0 )=67% of the tetrads have true tree structure. ( b ) Tree relationship among normal cell types based on discretized transcriptomic data using maximum parsimony method [21] . Colours indicate different groups of cells. Magenta: fibroblast and myoblast cells; cyan: immune cells; orange: epithelial cells; black: others. ( c ) Neighbour net [22] , [23] for the distance matrix for normal cells. Scale bar, 1,000. ( d ) Neighbour net of the distance matrix for neoplastic cells. Scale bar, 1,000. Note that the cancer cells have a greatly less resolved tree than normal cells, which is also reflected in the treeness statistic. Colour-marked samples are used for treeness test among cancer origin pairs. Full size image We next analysed the more extensive data of 127 normal human cell types from the FANTOM5 consortium. We proceeded in the same way as described above for the ENCODE data and calculated the α -value distribution for transcriptomes of normal cells. We again found evidence for extensive tree structure. Specifically, the data suggests that 50±5% of the tetrads have significant tree structure. Finally, we analysed 35 normal mouse cell types from FANTOM5 and found 74±5% of the tetrads has tree structure. The exact fraction of tetrads with tree structure varies between data sets, most probably reflecting differences in celltype sampling. Overall, these results support the notion that the transcriptomes of normal human and mouse cells have substantial tree structure, consistent with the sister cell-type model [4] ( Supplementary Fig. 1a,b ). Next, we took a look at those tetrads with significant low α -values. One thousand and six hundred out of 7,740 tetrads from the ENCODE normal human cells have α -values <0.05. In each tetrad with a tree structure, the four cell types are grouped into two pairs, as shown in Fig. 1d ( x , y ) and ( u , v ). Among these tetrads, some cell-type pairs are observed much more frequently than random expectation ( Supplementary Fig. 1c ), suggesting that these cell types are more closely related to each other and two randomly sampled cell types. For instance, mesenchymal cells are more frequently paired with other mesenchymal cells in tree-like tetrads than expected by chance. As the α -value distribution indicates extensive tree structure for those normal cell types, we built a phylogenetic tree of those samples using parsimony on the expression profile of protein-coding genes (for ENCODE data, see Fig. 2b,c ). It is clear that fibroblast and myoblast cells (magenta) aggregated together, immune cells (cyan) also aggregated together and epidermal cells (orange) from ectoderm form another cluster. Similar results are achieved with only transcription factor-coding genes. The rationale for analysing transcription factor gene expression separately is that the total similarity of total transcriptomes can be influenced by similarity of function rather than phylogenetic relationships. Similarly, immune cells are more frequently paired with other immune cells and so on, implying that the tree structure detected by our treeness test are biologically meaningful (for FANTOM5 data, see Supplementary Figs 2–3 ). Some samples probably represent the same cell type Cells analysed in this study have been designated as ‘different cell types’ based on their sampling location. For instance, there are a number of fibroblasts that have been sampled from different locations in the body, but it is not clear that they represent truly different cell types or just the same cell type in different parts of the body. We suggest that the ‘treeness test’ presented here can also be used as a first pass criterion to determine whether different samples could be from different cell types. In a comparison of two cell types, each represented by two replicates, one would expect that the replicates are more similar to each other than each replicate is to that of another cell type. Hence, tetrads consisting of two pairs of replicates from different cell types are expected to have significant tree structure ( Fig. 3a ). However, replicates that in fact are all from the same cell type will follow the null model and fail to reject the null hypothesis. This is in fact the case ( Fig. 3c ). In the comparison among skin and lung fibroblasts from human normal ENCODE cell samples the average α -values are marginal (median α -value=0.042), while for the comparison among all normal cell-type pairs we have lower α -values (median α -value=0.0091). This statistic shows that the fibroblasts from the skin and the lung are only marginally more different than two replicates of fibroblasts from the same location. FANTOM5 data show the same pattern ( Fig. 3d ), with fibroblast median α -value=0.049 and normal cells median α -value=0.017. This suggests that fibroblasts from different parts of the body could be the same cell type, even though their gene expression patterns might be slightly different due to modulation by local factors in the skin and the lung for instance. 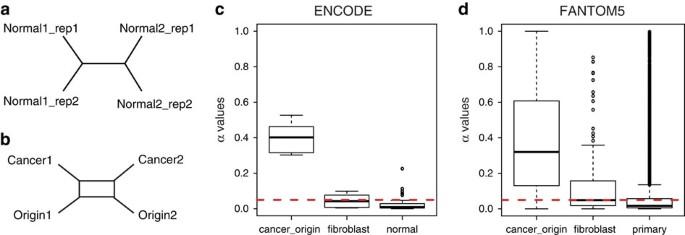Figure 3: Using the treeness test as a tool to identify distinct cell types. (a) Comparison of pairs of replicates between normal cell types. If the two cell samples are in fact two cell types, we expect the tetrad to have significant tree structure, meaning that replicates are more similar to each other than each is to a replicate from a different cell type. (b) To test whether cancer cells remain similar to their normal cell types from which they originate, we compare cancer cell transcriptomes with that of normal cell types from which the cancer originated, that is, each tetrad has two pairs, each consisting of a normal cell with their cognate cancer cell. (c) Results for ENCODE data. (d) Results for FANTOM5 data. Note that cancer cells are not more similar to their cells of origin than to unrelated cell types, indicating that cancer cells diverge more radically than novel cell types in evolution. Fibroblasts from different body parts have marginally significant tree structure, suggesting that they might be representing the same cell type in different locations of the body. Finally, replicates of the other normal cell types are highly significant, showing that their replicates are much more similar than they are to other cell types. In the box-and-whisker plot, the bottom and top of the box are the first and third quartiles. The ends of whiskers are the lowest datum still within 1.5 interquartile range of the lower quartile, and the highest datum within 1.5 interquartile range of the upper quartile. The red dotted line indicatesα=0.05. Figure 3: Using the treeness test as a tool to identify distinct cell types. ( a ) Comparison of pairs of replicates between normal cell types. If the two cell samples are in fact two cell types, we expect the tetrad to have significant tree structure, meaning that replicates are more similar to each other than each is to a replicate from a different cell type. ( b ) To test whether cancer cells remain similar to their normal cell types from which they originate, we compare cancer cell transcriptomes with that of normal cell types from which the cancer originated, that is, each tetrad has two pairs, each consisting of a normal cell with their cognate cancer cell. ( c ) Results for ENCODE data. ( d ) Results for FANTOM5 data. Note that cancer cells are not more similar to their cells of origin than to unrelated cell types, indicating that cancer cells diverge more radically than novel cell types in evolution. Fibroblasts from different body parts have marginally significant tree structure, suggesting that they might be representing the same cell type in different locations of the body. Finally, replicates of the other normal cell types are highly significant, showing that their replicates are much more similar than they are to other cell types. In the box-and-whisker plot, the bottom and top of the box are the first and third quartiles. The ends of whiskers are the lowest datum still within 1.5 interquartile range of the lower quartile, and the highest datum within 1.5 interquartile range of the upper quartile. The red dotted line indicates α =0.05. Full size image Transcriptomes of cancer cells have minimal tree structure Interestingly, for the cancerous cell types from ENCODE ( Supplementary Table 2 ), we arrived at a much lower fraction of tetrads with true tree structure, 1− π 0 =0.23, implying that only 23% of tetrads among neo-plastic cells have true tree structure ( Fig. 2d and Supplementary Fig. 1d ). The failure to find, among neoplastic cells, similar degrees of tree structure as with normal cells could be due to differences in the cell-type sampling. To further test whether this difference is biologically meaningful, we analysed tetrads with two normal cells (mammary epithelial cell and monocyte) and their derived cancer cells (mammary gland adenocarcinoma and leukemia cell) ( Fig. 3b ). If the cancer cells and their cells of origin are much more related to each other, the tetrad would have significant tree structure. However, if the origin of neoplastic cells is due to the recruitment of unrelated transcriptional modules, the tetrad would not have significant tree structure. This is actually the case as shown in Fig. 3c (median α -value=0.40 over tetrads with different replicates of these four cell samples). A very similar pattern is found in the FANTOM5 data, where the cancer cells compared with the cell types of origin have a median α -value of 0.32. This indicates that the relationships between normal cell types are lost on neoplastic transformation either through general downregulation of cell state-specific gene products or through the breakdown of correlated expression profiles caused by heterogeneous and independent genomic applications and deletions seen in different cancer genomes. Detecting significant tree structure in the transcriptomic data from a set of normal cell types has two broad implications. For one, it supports the sister cell-type model of cell origination in evolution [4] , and the second is that the analysis of cell-type trees can yield mechanistic insights. Here we briefly discuss these two points in turn. Although our results are consistent with the sister cell-type model, we note that the precise nature of this inference is a ‘failed attempt to falsify the sister cell-type model,’ in the sense of Karl Popper’s philosophy of science, rather than a conclusive proof, if conclusive proof is possible at all in the empirical sciences. If our results would have failed to find the tree structure, the sister cell-type model would have lost its standing as a probable model of cell-type evolution. We also note that the sister cell-type model predicts that closely related cell types have similar gene expression patterns, because they share the developmental trajectory that they inherited from their ancestral cell type. Hence, the sister cell-type model also predicts a degree of congruence between the similarity of transcriptomes (interpreted here as a phylogenetic signal) and the ontogenetic cell lineage relationships [4] . In our analysis, this is reflected in the transcriptomic similarity between macrophages and dendritic cells, which are both derived from monocytes, as well as the separation between lymphoid and myeloid cells, which represent separate ontogenetic cell lineages ( Supplementary Fig. 4 ) [14] but the congruence is limited probably because ontogenetic trajectories are to some degree flexible. The alternative to the sister cell-type model is analogous to hybridization of species. It would be a process where the new cell types arise by combining gene regulatory modules from very different cell types to create a new cell type. One consequence of this model is that new cell types do not arise as closely related and similar pairs. Naturally, under the ‘hybridization model’ of cell-type origination, the similarity structure among cell-type transcriptomes would be non-tree-like. In this context, it is interesting that we found substantially less tree structure among cancer cells, even when compared with their normal cell types of origin for each cancer ( Fig. 3 ). This finding suggests that tumorigenesis is associated with transcriptional dysregulation, rather than an orderly hierarchical differentiation process. The second consequence of our result is that the phylogenetic analysis of cell-type transcriptomes can allow biologically meaningful inferences, rather than just arbitrary classifications. Cell-type trees are hypotheses of the phylogenetic relationships among the cell types, similar to character trees as suggested by Oakley et al. [15] , [16] and Geeta [17] for plant parts. Consequently, phylogenetic reconstruction of ancestral transcriptomes, using standard phylogenetic methods, can reveal the history of gene recruitment events associated with the origin of a novel cell type in evolution and can lead to testable hypotheses about the molecular mechanisms of cell-type origination. Data processing RNA-seq data used in this analysis is from ENCODE [5] (available at http://hgdownload.cse.ucsc.edu/goldenPath/hg19/encodeDCC/wgEncodeCshlLongRnaSeq/ ). Samples are selected by ‘extraction method=longPolyA’ and ‘localization=cell’. Raw sequencing data are downloaded and aligned with Tophat [18] (version 2.0.6) to UCSC hg19. HTSeq [19] (version 0.6.1p1) is used to count reads with Ensembl [20] gene assembly Homo sapiens GRCh37.73. The tpm value for each gene is calculated based on read counts. A threshold of tpm=3 is used to discretize the tpm values. CAGE data used in this analysis is generated by FANTOM5 (ref. 7 ; available at http://fantom.gsc.riken.jp/5/data/ ). Only differentiated and not externally treated cell samples are selected for the treeness test. Expression table with tpm values for refSeq genes is downloaded and a threshold of tpm=2 is used to get the discretized expression profile. Derivation of null model δ -value distribution A full derivation of the null model δ distribution is available in Supplementary Methods ( Supplementary Figs 5 and 6 , and Supplementary Table 3 ). How to cite this article: Liang, C. et al. The statistical geometry of transcriptome divergence in cell-type evolution and cancer. Nat. Commun. 6:6066 doi: 10.1038/ncomm7066 (2015).